MPP8 mediates the interactions between DNA methyltransferase Dnmt3a and H3K9 methyltransferase GLP/G9a DNA CpG methylation and histone H3 lysine 9 (H3K9) methylation are two major repressive epigenetic modifications, and these methylations are positively correlated with one another in chromatin. Here we show that G9a or G9a-like protein (GLP) dimethylate the amino-terminal lysine 44 (K44) of mouse Dnmt3a (equivalent to K47 of human DNMT3A) in vitro and in cells overexpressing G9a or GLP. The chromodomain of MPP8 recognizes the dimethylated Dnmt3aK44me2. MPP8 also interacts with self-methylated GLP in a methylation-dependent manner. The MPP8 chromodomain forms a dimer in solution and in crystals, suggesting that a dimeric MPP8 molecule could bridge the methylated Dnmt3a and GLP, resulting in a silencing complex of Dnmt3a–MPP8–GLP/G9a on chromatin templates. Together, these findings provide a molecular explanation, at least in part, for the co-occurrence of DNA methylation and H3K9 methylation in chromatin. Both components of chromatin (DNA and histones) are subject to dynamic post-synthetic covalent modifications. DNA methylation is associated with histone modifications, particularly the demethylated state of histone H3 lysine 4 (H3K4me0) [1] and the methylated state of histone H3 lysine 9 (H3K9me) [2] . The functional linkage of DNA methylation, H3K4 methylation and H3K9 methylation is illustrated by the finding that treatment with 5-aza-2′-deoxycytidine (5-aza), a DNA-demethylation drug [3] , leads to depletion of DNA methylation and of H3K9 methylation, and a corresponding increase in H3K4 methylation [4] . Furthermore, mono- and di-methylated H3K9 (H3K9me1/me2), the reaction products of G9a and G9a-like protein (GLP) [5] , [6] , are the silencing marks that are lost when tumour-suppressor genes—for example, in colorectal cancer cells [7] and in breast cancer cells [8] —are reactivated following treatment with 5-aza. Considering the inverse relationship between H3K4 methylation and DNA methylation, it is important that the mammalian lysine specific demethylases LSD1 and LSD2, which acts on di- and mono-methylated H3K4 (H3K4me2/me1), are absolutely essential for maintaining global DNA methylation (LSD1) [9] and establishing maternal DNA genomic imprints (LSD2) [10] . Indeed, disruption of LSD1 results in earlier embryonic lethality and a more severe DNA hypomethylation defect than the disruption of DNA methyltransferases themselves [9] . The de novo DNA methyltransferase Dnmt3a–Dnmt3L complex contains components for reading H3K4me0 (refs 1 , 11 ) and methylating DNA in regions of chromatin, where H3K4 is unmodified [12] . In contrast to that at H3K4, methylation at H3K9 is positively correlated with DNA methylation. There is in vivo evidence that the H3K9-linked DNA methylations represent an evolutionarily conserved silencing pathway. In Neuropora and Arabidopsis , DNA methylation is strictly dependent on the H3K9 methyltransferases [13] , [14] , [15] . With regard to mammals, G9a and GLP, two related euchromatin-associated H3K9 methyltransferases forming heterodimers [6] , have been implicated in DNA methylation at various loci, including imprinting centres [16] , [17] , retrotransposons and satellite repeats [18] , a G9a/GLP target promoter [19] , Oct4 promoter [20] , [21] , and a set of embryonic genes [22] . Furthermore, G9a is required for de novo DNA methylation and establishment of silencing of newly integrated proviruses in murine embryonic stem cells [23] . Here we study the physical interactions of G9a/GLP and de novo DNA methyltransferase Dnmt3a. We find that the amino-terminal lysine 44 of mouse Dnmt3a (equivalent to lysine 47 of human DNMT3A) is dimethylated by G9a/GLP. We also find that the resulting modification (Dnmt3aK44me2) is recognized by the chromodomain of MPP8 (M-phase phosphoprotein 8), a protein known to interact with both GLP and Dnmt3a in silencing E-cadherin gene [24] . The G9a/GLP–Dnmt3a–MPP8 methyl–lysine signalling network represents a molecular link between the mechanisms that establish DNA methylation and H3K9 methylation. Dimethylation of Dnmt3a at Lys44 by G9a/GLP Both Dnmt3a and G9a/GLP are multi-domain proteins [25] , [26] ( Fig. 1a ). Recent reports suggested that two very different regions of Dnmt3a, either the N-terminal regulatory domain [27] or the carboxy-terminal catalytic domain [22] , are involved in interaction with G9a. We first asked whether Dnmt3a could be a substrate of G9a or GLP enzymatic activities, as they have been shown to act on non-histone proteins [28] . Using various mouse Dnmt3a domain fragments ( Supplementary Fig. S1a ), we showed that G9a and GLP catalytic SET domains (named after three Drosophila proteins, s uppressor of variegation [Su(var)3-9], e nhancer of zeste [E(z)] and t rithorax [Trx]) methylate the N-terminal fragment of Dnmt3a (Dnmt3a-N) in vitro ( Supplementary Fig. S1b ). Although Dnmt3a and Dnmt3b have similar domain arrangements, their N-terminal sequences share no similarity, and only Dnmt3a is modified by G9a and GLP ( Fig. 1b ; Supplementary Fig. S1c ). To identify methylation site(s), we carried out the methylation experiments for various lengths of time, isolated the methylated Dnmt3a-N and analysed the peptide fragments by MALDI mass spectrometry. Only the fragment corresponding to residues 35–58 had mass additions, corresponding to mono- and di-methylation ( Fig. 1c ). Although this fragment contains three potential methylation sites, K44, K51, and K53, we suspected K44 as the major site, because the amino-side sequences adjacent to mDnmt3a K44 and histone H3K9 (a known substrate of G9a) are the same TARK tetrapeptide ( Fig. 1a ). To test this, we showed that introducing a K44R mutation eliminates methylation ( Fig. 1b ; Supplementary Fig. S1d ). Furthermore, parallel experiments with human DNMT3A identified K47 (equivalent to K44 of mDnmt3a; Fig. 1a ) as the only methylation site for GLP in vitro ( Fig. 1d–f ). As negative controls, neither H3K9 methyltransferase Suv39, nor any of three other known protein lysine methyltransferases, methylate Dnmt3a in vitro ( Supplementary Fig. S2a ). 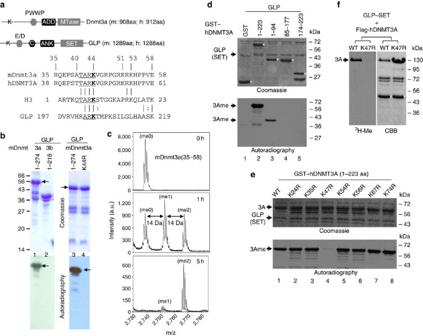Figure 1: Dnmt3a is dimethylated by GLPin vitro. (a) Dnmt3a and GLP domain arrangements (h: human; m: mouse). Underlining indicates the shared TARK sequence motif that includes K44 of mDNMT3a, K47 of hDNMT3A, and K9 of histone H3. (b) The N-terminal domain of mDnmt3a (residues 1–274) is methylated (lanes 1 and 3). The methylation reaction was carried out with [3H]-AdoMet and analysed by fluorography. The N-terminal domain of mDnmt3b is not methylated (lane 2). A K44R substitution in mDnmt3a eliminates methylation (lane 4). (c) Mass spectrometry of the products ofin vitromethylation assays (0 h, preincubation; 1 and 5 h, after reaction) after isolating the methylated mDnmt3a (residues 1–274) from SDS-gel, performing in-gel digestion with V8 protease, and analysing the peptide fragments by MALDI mass spectrometry. The mass shift of 14 Da represents addition of one methyl group. (d) Gel image (top) and autoradiogram (bottom) ofin vitromethylation assays with His-GLP-catalytic SET domain on various GST-tagged hDNMT3A N-terminal fragments (labelled with *) with residue numbers indicated. The N-terminal fragments of hDNMT3A (residues 1–223 and 1–94) are methylated (lanes 2 and 3). (e) K47R substitution in hDNMT3A N-terminal domain (residues 1–223) eliminates methylation (lane 4). (f) K47R substitution in hDNMT3A, in the context of full-length protein, eliminates methylation. Figure 1: Dnmt3a is dimethylated by GLP in vitro . ( a ) Dnmt3a and GLP domain arrangements (h: human; m: mouse). Underlining indicates the shared TARK sequence motif that includes K44 of mDNMT3a, K47 of hDNMT3A, and K9 of histone H3. ( b ) The N-terminal domain of mDnmt3a (residues 1–274) is methylated (lanes 1 and 3). The methylation reaction was carried out with [ 3 H]-AdoMet and analysed by fluorography. The N-terminal domain of mDnmt3b is not methylated (lane 2). A K44R substitution in mDnmt3a eliminates methylation (lane 4). ( c ) Mass spectrometry of the products of in vitro methylation assays (0 h, preincubation; 1 and 5 h, after reaction) after isolating the methylated mDnmt3a (residues 1–274) from SDS-gel, performing in-gel digestion with V8 protease, and analysing the peptide fragments by MALDI mass spectrometry. The mass shift of 14 Da represents addition of one methyl group. ( d ) Gel image (top) and autoradiogram (bottom) of in vitro methylation assays with His-GLP-catalytic SET domain on various GST-tagged hDNMT3A N-terminal fragments (labelled with *) with residue numbers indicated. The N-terminal fragments of hDNMT3A (residues 1–223 and 1–94) are methylated (lanes 2 and 3). ( e ) K47R substitution in hDNMT3A N-terminal domain (residues 1–223) eliminates methylation (lane 4). ( f ) K47R substitution in hDNMT3A, in the context of full-length protein, eliminates methylation. Full size image We further investigated whether Dnmt3a is methylated by G9a or GLP in vivo . As an initial step, Flag-tagged Dnmt3a was coexpressed with G9a or GLP in human embryonic kidney 293T cells, and then immunoprecipitated with anti-Flag antibody for western blot analysis using an anti-pan methyl–lysine antibody ( Supplementary Fig. S2b ). The results indicate that G9a and GLP are associated with Dnmt3a methylation in cells ( Supplementary Fig. S2b ). We then stably knocked-down GLP in 293T cells using vector-based short hairpin RNA (>90% efficiency at protein level, Supplementary Fig. S3a ). Myc-hDNMT3A (WT or the methylation-deficient K47R mutant) was then coexpressed with GLP or G9a in these cells for metabolic labelling (via 3 H-Met) [29] . The autoradiograph of Myc-immunoprecipitated protein indicates that the level of 3 H-labelled hDNMT3A is markedly increased in cells co-transfected with wild-type GLP or G9a expression vector, but not in cells coexpressing enzymatic inactive GLP mutant C1203A nor in the hDNMT3A mutant K47R that cannot be methylated ( Fig. 2a ). These results are consistent with GLP and G9a methylating hDNMT3A at K47 in vivo . Furthermore, mass spectrometric analysis of hDNMT3A, immunoprecipitated from 293T cells co-transfected with wild-type GLP and hDNMT3A, independently revealed in vivo mono- and dimethylation at K47 of hDNMT3A ( Fig. 2b ). 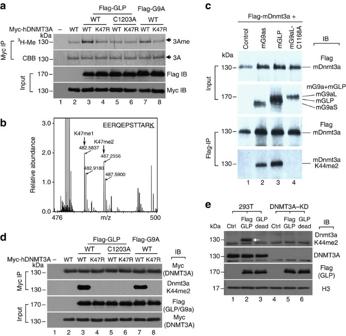Figure 2: Dnmt3a is methylated in cells by overexpressing GLP or G9a. (a) hDNMT3A-WT or K47R mutant was coexpressed with GLP (WT or C1203A mutant) or G9a inGLPknockdown 293T cells for metabolic labelling with [methyl-3H]-Met (ref.29). After Myc-immunoprecipitation, methylated-hDNMT3A is visualized by autoradiogram. (b) Myc-hDNMT3A was coexpressed with Flag-GLP in 293T cell, purified by Myc-IP and digested after SDS–PAGE for tandem mass spectrometry (LC-MS/MS) analysis. Mono- and di-methylation of K47 were detected. (c) Flag-tagged mDnmt3a was overexpressed together with mouse G9a (lane 2), or mouse GLP (lane 3), or a G9a catalytic dead mutant (lane 4) in 293T cells. Flag-tagged mDnmt3a was immunoprecipitated by anti-Flag antibody and subjected to western blot analysis by anti-mDnmt3aK44me2 antibody. (d) hDNMT3A-WT or K47R mutant was coexpressed with GLP or G9a inGLPknockdown 293T cells for IP-western analysis. Methylated-hDNMT3A is detected by anti-mDnmt3aK44me2 antibody (lanes 3 and 7). (e) Overexpressing GLP methylates endogenous Dnmt3a (indicated by the white arrow). Flag-GLP–WT or C1203A mutant (GLP dead) was expressed in control (lanes 1–3) orDNMT3Aknockdown 293T cells (lanes 4–6). Nuclear pellet fraction was examined by western blot using indicated antibodies. Figure 2: Dnmt3a is methylated in cells by overexpressing GLP or G9a. ( a ) hDNMT3A-WT or K47R mutant was coexpressed with GLP (WT or C1203A mutant) or G9a in GLP knockdown 293T cells for metabolic labelling with [methyl- 3 H]-Met (ref. 29 ). After Myc-immunoprecipitation, methylated-hDNMT3A is visualized by autoradiogram. ( b ) Myc-hDNMT3A was coexpressed with Flag-GLP in 293T cell, purified by Myc-IP and digested after SDS–PAGE for tandem mass spectrometry (LC-MS/MS) analysis. Mono- and di-methylation of K47 were detected. ( c ) Flag-tagged mDnmt3a was overexpressed together with mouse G9a (lane 2), or mouse GLP (lane 3), or a G9a catalytic dead mutant (lane 4) in 293T cells. Flag-tagged mDnmt3a was immunoprecipitated by anti-Flag antibody and subjected to western blot analysis by anti-mDnmt3aK44me2 antibody. ( d ) hDNMT3A-WT or K47R mutant was coexpressed with GLP or G9a in GLP knockdown 293T cells for IP-western analysis. Methylated-hDNMT3A is detected by anti-mDnmt3aK44me2 antibody (lanes 3 and 7). ( e ) Overexpressing GLP methylates endogenous Dnmt3a (indicated by the white arrow). Flag-GLP–WT or C1203A mutant (GLP dead) was expressed in control (lanes 1–3) or DNMT3A knockdown 293T cells (lanes 4–6). Nuclear pellet fraction was examined by western blot using indicated antibodies. Full size image We next raised an antibody to the mDnmt3aK44me2 epitope. The affinity-purified anti-mDnmt3aK44me2 antibody specifically recognized mDnmt3aK44me2 peptides but not unmodified peptides ( Supplementary Fig. S2c ). This antibody detects mDnmt3a–K44me2 robustly in Flag-mDnmt3a, immunoprecipitated from 293T cells coexpressing G9a or GLP ( Fig. 2c ), but not coexpressing the inactive G9a mutant ( Fig. 2c ; Supplementary Fig. S2b ). The same antibody recognized Myc-hDNMT3A coexpressed with G9a or GLP in GLP stable knockdown cells ( Fig. 2d ), but not with GLP catalytic inactive mutant C1203A [19] ( Fig. 2d ), nor with the hDNMT3A non-methylatable K47R mutant ( Fig. 2d ). Next, we asked whether G9a/GLP methylates endogenous Dnmt3a. Dnmt3a is expressed at a low level in most somatic cells [30] , and associates tightly with nucleosomes [31] , [32] , as it is found mainly in the nuclear pellet fraction [27] ( Supplementary Fig. S3b ). Western blot analysis of the nuclear pellet fraction derived from 293T cells [33] , [34] did not detect hDNMT3A–K47 methylation (by anti-mDnmt3aK44me2) ( Fig. 2e ), suggesting the amount of this form is too low to be detected. However, K47 methylation of endogenous hDNMT3A was readily detectable in cells expressing GLP-WT ( Fig. 2e ) but not in cells either expressing the GLP catalytically inactive mutant ( Fig. 2e ) or in DNMT3A stable knockdown 293T cells ( Fig. 2e ; Supplementary Fig. S3c ). Structure of the GLP–Dnmt3a peptide complex To understand the molecular basis of Dnmt3a methylation catalyzed by G9a and GLP, we first measured the dissociation constant ( K D ) for the interaction between the unmodified mDnmt3a(39–50)K44me0 peptide substrate and G9a or GLP catalytic SET domains. The affinities are in the range of 4–6 μM ( Fig. 3a ). The same mDnmt3a peptide encompassing amino acids 39–50 was used for co-crystallization with GLP SET domain in the presence of the methyl donor analogue Sinefungin (adenosyl ornithine) ( Supplementary Table S1 ). 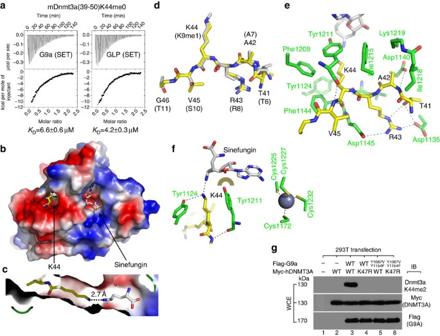Figure 3: Structure of GLP–Dnmt3a complex. (a) ITC measurement of binding of G9a (left) or GLP (right) SET domain to unmodified mDnmt3aK44me0 peptide in the presence of one of the reaction products S-adenosyl-L-homocysteine (to prevent the enzymatic reaction as well as the release of the substrate). (b) The substrate peptide and the methyl donor analogue Sinefungin bind in two distinctive binding sites in the opposite ends of a narrow target-lysine channel (see panelc). (c) The AdoMet analogue sinefungin (adenosyl ornithine) was used to prepare the ternary complex. This mimics the step before methyl transfer, because sinefungin also carries a formal positive charge on the ɛ-amino group (N+-C in the place of C-S+of AdoMet). The target amino group of lysine K44 and the ɛ-amino group of sinefungin are in near linear conformation (N•••N distance of 2.7 Å and N•••N–C angle of 165°). (d) Superimposition of mDnmt3a peptide (yellow) and H3K9 peptide (grey) bound with GLP SET domain (derived from PDB 3HNA35). The nitrogen atoms are in blue, the oxygen atoms in red, and the carbon atoms in yellow (mDnmt3a) or grey (H3). (e) Electrostatic interactions, hydrogen bonds (dashed lines) and van der Waals interactions define GLP–mDnmt3a peptide interactions. mDnmt3a-R43 bridges between GLP–Asp1135 and GLP–Asp1145. GLP–Asp1135 hydrogen bonds with the side-chain hydroxyl oxygen atom of mDnmt3a-T41, which in turn makes an intra-molecular interaction with mDnmt3a-R43. mDnmt3a-A42 fits into a shallow hydrophobic pocket formed by Ile1218, Phe1215, and the aliphatic portion of Lys1219 of GLP. (f) Two tyrosines, Tyr 1124 and Tyr1211 (GenBank CAH71077.1), flank the target lysine K44 of mDnmt3a. (g) The corresponding tyrosines in human G9a are Y1067 and Y1154 (NCBI NP_006700.3). Coexpression of the G9a double mutant (Y1067V/Y1154F) and hDNMT3A in 293T cells failed to methylate K47 (lane 5). The whole-cell extract was analysed by western blot using the indicated antibodies. Figure 3: Structure of GLP–Dnmt3a complex. ( a ) ITC measurement of binding of G9a (left) or GLP (right) SET domain to unmodified mDnmt3aK44me0 peptide in the presence of one of the reaction products S-adenosyl-L-homocysteine (to prevent the enzymatic reaction as well as the release of the substrate). ( b ) The substrate peptide and the methyl donor analogue Sinefungin bind in two distinctive binding sites in the opposite ends of a narrow target-lysine channel (see panel c ). ( c ) The AdoMet analogue sinefungin (adenosyl ornithine) was used to prepare the ternary complex. This mimics the step before methyl transfer, because sinefungin also carries a formal positive charge on the ɛ-amino group (N + -C in the place of C-S + of AdoMet). The target amino group of lysine K44 and the ɛ-amino group of sinefungin are in near linear conformation (N•••N distance of 2.7 Å and N•••N–C angle of 165°). ( d ) Superimposition of mDnmt3a peptide (yellow) and H3K9 peptide (grey) bound with GLP SET domain (derived from PDB 3HNA [35] ). The nitrogen atoms are in blue, the oxygen atoms in red, and the carbon atoms in yellow (mDnmt3a) or grey (H3). ( e ) Electrostatic interactions, hydrogen bonds (dashed lines) and van der Waals interactions define GLP–mDnmt3a peptide interactions. mDnmt3a-R43 bridges between GLP–Asp1135 and GLP–Asp1145. GLP–Asp1135 hydrogen bonds with the side-chain hydroxyl oxygen atom of mDnmt3a-T41, which in turn makes an intra-molecular interaction with mDnmt3a-R43. mDnmt3a-A42 fits into a shallow hydrophobic pocket formed by Ile1218, Phe1215, and the aliphatic portion of Lys1219 of GLP. ( f ) Two tyrosines, Tyr 1124 and Tyr1211 (GenBank CAH71077.1), flank the target lysine K44 of mDnmt3a. ( g ) The corresponding tyrosines in human G9a are Y1067 and Y1154 (NCBI NP_006700.3). Coexpression of the G9a double mutant (Y1067V/Y1154F) and hDNMT3A in 293T cells failed to methylate K47 (lane 5). The whole-cell extract was analysed by western blot using the indicated antibodies. Full size image Like all structurally characterized SET domain proteins, the mDnmt3a peptide binds to a surface groove of the SET domain ( Fig. 3b ) with the target lysine mDnmt3a-K44 inserted into a narrow aromatic channel, such that the target nitrogen lies in close proximity to the methyl donor analogue at the opposite end ( Fig. 3c ). The mDnmt3a peptide specificity is determined primarily through recognition of ordered side chains of T41-A42-R43 and V45-G46, residues before and after the target lysine K44, respectively (one letter-code used for mDnmt3a residues). The Dnmt3a peptide conformation is nearly identical with that of histone H3 peptide bound with GLP SET domain [35] ( Fig. 3d ). The network of interactions involves electrostatic salt bridges, hydrogen bonds and van der Waals contacts ( Fig. 3e ). The side chain of target lysine K44 bound in a narrow aromatic channel with aromatic side chains of GLP (Tyr1124, Phe1144, Phe1209, Tyr1211 and Phe1215) wrapping around its aliphatic chain (three-letter code used to distinguish GLP residues). The terminal amino group of substrate target K44 hydrogen bonds with the hydroxyl oxygen atom of Tyr1124 ( Fig. 3f ). The corresponding Y178V mutation in DIM-5 (a Neurospora H3K9 methyltransferase) caused complete loss of its enzymatic activity [36] . The hydroxyl group of Tyr1211 of GLP is hydrogen-bonded to the backbone carbonyl oxygen of Ile1168 (not shown) and is in van der Waals contact with the ribose and adenine rings of Sinefungin ( Fig. 3f ). The corresponding Y283F mutation in DIM-5 lost AdoMet binding and thus activity [37] . The formation of the aromatic channel coincides with the 'post-SET' zinc binding by four cysteines (Cys1172, Cys1225, Cys1227 and Cys1232) near the cofactor-binding site ( Fig. 3f ), which is required for activity of DIM-5 (ref. 37 ). The complex structure of GLP–mDnmt3a–sinefungin thus predicted that mutations occurring to side chains of GLP–C1172A (GenBank accession codes CAH71077.1 or C1203A of NP_079033.4, as in Fig. 2a and Fig. 2d ) or G9a–Y1067V and G9a–Y1154F ( Fig. 3g ) would affect Dnmt3a methylation by GLP or G9a, respectively. MPP8 chromodomain is a Dnmt3aK44me2 reader domain Besides the catalytic SET domain, G9a and GLP also contain methyl–lysine binding ankyrin repeats [38] , [39] . These can bind H3K9me2/me1, the reaction products of the G9a/GLP catalytic domain [38] . However, the ankyrin-repeat domain of GLP does not bind Dnmt3a(39–50) peptide either dimethylated or unmodified at K44 ( Supplementary Fig. S4a ). To understand the molecular basis of the function associated with Dnmt3aK44me2, we screened CADOR microarrays [40] for protein domains that might act as readers of this mark ( Supplementary Fig. S4b ). Of the 268 proteins on the array, the Dnmt3aK44me2 peptide can be recognized by a few potential readers, among them the chromodomain of MPP8. We focused on MPP8, because it was already shown to interact with GLP and Dnmt3a in modulating the expression of E-cadherin [24] . Measurement of dissociation constants independently confirmed direct interaction between the chromodomain of MPP8 and mDnmt3aK44me2, with a K D of ∼ 12 μM ( Fig. 4a ). 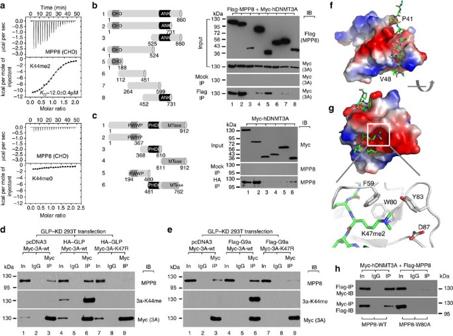Figure 4: MPP8 recognizes methylated Dnmt3a. (a) ITC measurement of binding of the MPP8 chromodomain to mDnmt3a peptide with (top) and without (bottom) K44me2 methylation. (b) The chromodomain of MPP8 is sufficient to interact with hDNMT3A. Various domains of MPP8 are indicated at left of the panels with a schematic presentation of the Flag-MPP8 constructs. Different MPP8 deletions were coexpressed with full-length Myc-hDNMT3A in 293T cells for immunoprecipitation–western analysis using various antibodies. (c) The N-terminal domain of hDNMT3A associates with endogenous MPP8. Schematic representation shows Myc-hDNMT3A deletion proteins with numbers indicate amino-acid positions (left). The 293T cells transiently transfected with plasmids encoding various Myc-hDNMT3A proteins. Cell lysates were immunoprecipitated with anti-Myc antibody. and western blot was carried out using anti-Myc or MPP8 antibodies (right). (d) K47 methylation stimulates MPP8-hDNMT3A interaction in cells. Myc-hDNMT3A (WT or K47R mutant) was coexpressed with HA–GLP inGLPstable knockdown 293T cells. After Myc-IP, western blot using indicated antibodies analysed methylation of hDNMT3A and its interaction with co-precipitated endogenous MPP8. In, 1% input. (e) Myc-hDNMT3A (WT or K47R mutant) was coexpressed with Flag-G9a inGLPstable knockdown 293T cells (In, 1% input). (f) Monomer structure of MPP8 chromodomain (in surface representation displayed in blue for positive, red for negative and white for neutral) bound to a peptide of hDNMT3AK47me2 (in stick model coloured green). (g) K47me2 of hDNMT3A binds in a partial hydrophobic cage of MPP8 formed by three aromatic residues (Phe59, Trp80 and Tyr83) and one aspartate (Asp87). One of its terminalN-CH3groups projects towards the three aromatic rings, whereas the second methyl group points towards Asp87, a typical arrangement of methyl–lysine binding cage52. (h) Substitution of the cage-forming residue (W80A) impairs MPP8 interactions with hDNMT3A. Flag-MPP8-WT or W80A mutant was coexpressed with Myc-hDNMT3A inMPP8stably knockdown 293T cells. Immunoprecipitation–western analyses were carried out using the antibodies indicated. Cell lysates were briefly sonicated followed by micrococcal nuclease treatments before immunoprecipitation to release chromatin-bound proteins. In, 2% input. Figure 4: MPP8 recognizes methylated Dnmt3a. ( a ) ITC measurement of binding of the MPP8 chromodomain to mDnmt3a peptide with (top) and without (bottom) K44me2 methylation. ( b ) The chromodomain of MPP8 is sufficient to interact with hDNMT3A. Various domains of MPP8 are indicated at left of the panels with a schematic presentation of the Flag-MPP8 constructs. Different MPP8 deletions were coexpressed with full-length Myc-hDNMT3A in 293T cells for immunoprecipitation–western analysis using various antibodies. ( c ) The N-terminal domain of hDNMT3A associates with endogenous MPP8. Schematic representation shows Myc-hDNMT3A deletion proteins with numbers indicate amino-acid positions (left). The 293T cells transiently transfected with plasmids encoding various Myc-hDNMT3A proteins. Cell lysates were immunoprecipitated with anti-Myc antibody. and western blot was carried out using anti-Myc or MPP8 antibodies (right). ( d ) K47 methylation stimulates MPP8-hDNMT3A interaction in cells. Myc-hDNMT3A (WT or K47R mutant) was coexpressed with HA–GLP in GLP stable knockdown 293T cells. After Myc-IP, western blot using indicated antibodies analysed methylation of hDNMT3A and its interaction with co-precipitated endogenous MPP8. In, 1% input. ( e ) Myc-hDNMT3A (WT or K47R mutant) was coexpressed with Flag-G9a in GLP stable knockdown 293T cells (In, 1% input). ( f ) Monomer structure of MPP8 chromodomain (in surface representation displayed in blue for positive, red for negative and white for neutral) bound to a peptide of hDNMT3AK47me2 (in stick model coloured green). ( g ) K47me2 of hDNMT3A binds in a partial hydrophobic cage of MPP8 formed by three aromatic residues (Phe59, Trp80 and Tyr83) and one aspartate (Asp87). One of its terminal N -CH 3 groups projects towards the three aromatic rings, whereas the second methyl group points towards Asp87, a typical arrangement of methyl–lysine binding cage [52] . ( h ) Substitution of the cage-forming residue (W80A) impairs MPP8 interactions with hDNMT3A. Flag-MPP8-WT or W80A mutant was coexpressed with Myc-hDNMT3A in MPP8 stably knockdown 293T cells. Immunoprecipitation–western analyses were carried out using the antibodies indicated. Cell lysates were briefly sonicated followed by micrococcal nuclease treatments before immunoprecipitation to release chromatin-bound proteins. In, 2% input. Full size image Independently, we mapped the interactions of MPP8 with hDNMT3A through co-immunoprecipitation of serial deletion mutants transiently expressed in 293T cells. We determined that the N-terminal 188 amino acids of MPP8, including the chromodomain, are sufficient to interact with hDNMT3A ( Fig. 4b ), whereas the N-terminal region of hDNMT3A, including the lysine residue K47, interacts with endogenous MPP8 ( Fig. 4c ). To further determine the importance of K47 methylation in hDNMT3A–MPP8 interaction in vivo , we coexpressed Myc-hDNMT3A-WT, or its K47R mutant with GLP in GLP stable knockdown 293T cells, and examined associations of different hDNMT3A with endogenous MPP8 by immunoprecipitation–western analyses. No K47 methylation was detected (by anti-mDnmt3aK44me2) when hDNMT3A was expressed alone in cells, and hDNMT3A interacted with MPP8, although weakly ( Fig. 4d ). When coexpressed with GLP, hDNMT3A was heavily methylated at K47, and the hDNMT3A–MPP8 interaction was significantly strengthened ( Fig. 4d ). On the contrary, non-methylatable hDNMT3A–K47R did not pull down endogenous MPP8, even when it was coexpressed with GLP ( Fig. 4d ). Similarly K47 methylation-dependent hDNMT3A–MPP8 interaction was also observed when hDNMT3A was coexpressed with G9a ( Fig. 4e ). These results demonstrate that K47 and its methylation mediate hDNMT3A–MPP8 interaction in vivo . Finally, we determined the structure of MPP8 chromodomain in complex with hDNMT3AK47me2 peptide (amino acids 40–53) ( Fig. 4f ; Supplementary Table S1 ). The hDNMT3A peptide bound in an extended conformation in an acidic cleft of the chromodomain ( Fig. 4f ). The isolated chromodomain interacts with eight hDNMT3A residues from P41–V48, with major interactions occurring N-terminal to the dimethylated K47 ( Fig. 5 ). In comparison, the ankyrin repeat domain of GLP binds H3K9me2 peptide with specific interactions to the residues (particularly S10 of H3) C-terminal to the dimethylated H3K9 (ref. 38 ), rendering it inert in binding the methylated Dnmt3a. The dimethylated K47 is bound in a partial hydrophobic and open cage formed by three aromatic residues (Phe59, Trp80 and Tyr83) and one acidic residue (Asp87) of MPP8 ( Fig. 4g ). Mutation of Trp80 to alanine (W80A) abrogate binding to hDNMT3a when they were coexpressed in MPP8 stable knockdown 293T cells [24] ( Fig. 4h ). Taken together, these results suggest that hDNMT3A–MPP8 interaction is mediated in a methylation-dependent manner by GLP-catalyzed hDNMT3A–K47 methylation. 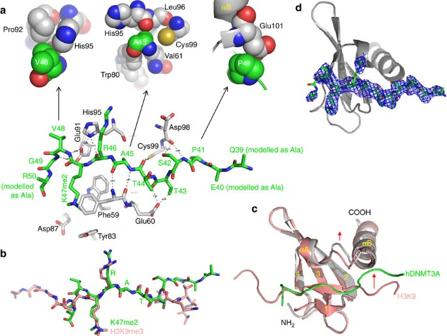Figure 5: Comparison of MPP8 chromodomain structures bound with hDNMT3AK47me2 and H3K9me3 peptides. (a) Binding specificity of hDNMT3AK47me2 peptide by MPP8. Stick model showing the hDNMT3A peptide (green), residues 39–50 (out of the residues 39–53 used for crystallization). The side chains of resides 39, 40 and 50 were modelled as alanines, whereas residues 51–53 were disordered. The MPP8 chromodomain contacts the eight residues (P41–V48) of the hDNMT3A peptide via hydrogen bonds (dashed lines) and van der Waals contact with P41, A45 and V48 (shown, respectively, in space-filling model). (b) Superimposition of hDNMT3AK47me2 peptide (green) and H3K9me3 peptide (orange) bound with MPP8 chromodomain (derived from PDB 3QO2 (ref.44)). The conformations of the conserved TARK tetrapeptide sequence overlaps well in the two structures, whereas the residues away from the conserved sequence adopt different conformations. The largest difference lies in the N-terminal residues of bound hDNMT3 with a bent conformation at P41–S42, whereas the H3 peptide exhibited an extended conformation. (c) Superimposition of MPP8-hDNMT3AK47me2 structure (protein in grey and peptide in green) with that of MPP8-H3K9me3 (orange). The pairwise root-mean-square-deviation between the two structures is∼0.6 Å (54 pairs of main-chain atoms). The MPP8 loop between helices αA and αB undergoes a concerted movement (as indicated by a red arrow) along with the different peptide conformations observed in panelb. The loop includes residue Asp98 interacting with S42 of hDNMT3A (see panela). The β strands are labelled by numbers. (d) Omit electron density, 2Fo–Fc, contour at 1σabove the mean, is superimposed with the refined K47me2 peptide. Figure 5: Comparison of MPP8 chromodomain structures bound with hDNMT3AK47me2 and H3K9me3 peptides. ( a ) Binding specificity of hDNMT3AK47me2 peptide by MPP8. Stick model showing the hDNMT3A peptide (green), residues 39–50 (out of the residues 39–53 used for crystallization). The side chains of resides 39, 40 and 50 were modelled as alanines, whereas residues 51–53 were disordered. The MPP8 chromodomain contacts the eight residues (P41–V48) of the hDNMT3A peptide via hydrogen bonds (dashed lines) and van der Waals contact with P41, A45 and V48 (shown, respectively, in space-filling model). ( b ) Superimposition of hDNMT3AK47me2 peptide (green) and H3K9me3 peptide (orange) bound with MPP8 chromodomain (derived from PDB 3QO2 (ref. 44 )). The conformations of the conserved TARK tetrapeptide sequence overlaps well in the two structures, whereas the residues away from the conserved sequence adopt different conformations. The largest difference lies in the N-terminal residues of bound hDNMT3 with a bent conformation at P41–S42, whereas the H3 peptide exhibited an extended conformation. ( c ) Superimposition of MPP8-hDNMT3AK47me2 structure (protein in grey and peptide in green) with that of MPP8-H3K9me3 (orange). The pairwise root-mean-square-deviation between the two structures is ∼ 0.6 Å (54 pairs of main-chain atoms). The MPP8 loop between helices αA and αB undergoes a concerted movement (as indicated by a red arrow) along with the different peptide conformations observed in panel b . The loop includes residue Asp98 interacting with S42 of hDNMT3A (see panel a ). The β strands are labelled by numbers. ( d ) Omit electron density, 2Fo–Fc, contour at 1 σ above the mean, is superimposed with the refined K47me2 peptide. Full size image MPP8 chromodomain binds self-methylated GLP Interestingly, G9a and GLP are auto-methylated in their N-terminal regions [28] , [41] , [42] . An N-terminal fragment of GLP (GLP–N, residues 191–280) containing K205 (which shares ARK sequence with that of K47 of hDNMT3a, Fig. 1a ) is methylated in vitro by recombinant GLP–SET domain, whereas the K205R substitution completely abolishes this GLP-catalyzed methylation ( Fig. 6a ). We next asked whether MPP8 could also bind to GLP methylated at K205. Recombinant GLP–N proteins (WT or the methylation deficient K205R mutant) were incubated with GLP catalytic SET domain for in vitro methylation and then immobilized on glutathione beads. Using in vitro translated MPP8 for GST pull-down, a robust direct interaction between GLP–N and MPP8 was observed only when K205 methylation occurs ( Fig. 6b ). The same GLP–N fragment, either unmethylated or containing K205R mutation, completely lost the interaction with MPP8 in the same assay. 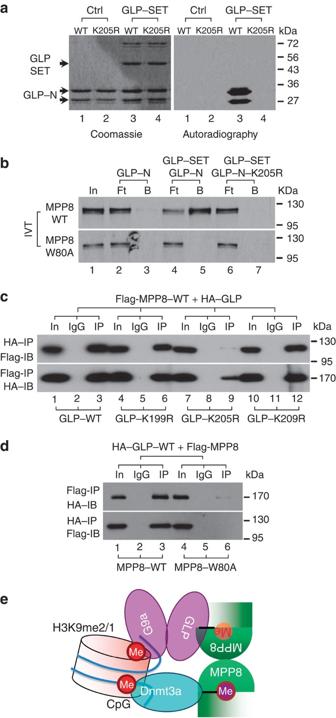Figure 6: MPP8 binds self-methylated GLP. (a) GLP self-methylates lysine residue at K205. Wild-type (WT) or K205R mutated GST–GLP–N terminal fragment (residues 191–280) was incubated with (lanes 3–4) or without (lanes 1–2) His–GLP–SET domain (residues 955–1,298) for methylation assays. Auto-radiogram (right) shows methylation. (b) MPP8 binds to methylated GLP at K205in vitro. GST–GLP–N–WT or its K205R mutant in the context of fragment 191–280 was incubated with His–GLP–SET domain forin vitromethylation. After being purified and immobilized on glutathione beads, GST–GLP–N terminal fragment was incubated within vitrotranslated FL-35S–MPP8–WT (top panel) or its W80A mutant (bottom panel) for GST pull-down. Label 'B' indicates the bound fraction and 'Ft' the flow through. In, 5% input. (c) MPP8–GLP interaction is mediated through GLP–K205 in cells. Flag-MPP8-WT was coexpressed with HA-GLP–WT, K199R, K205R or K209R mutant in 293T cells. Cell lysates were immunoprecipitated with anti-HA (top panel) or Flag (bottom panel) antibody. Co-immunoprecipitated Flag-MPP8 or HA–GLP were analysed by western blot using indicated antibodies. In, 5% input. (d) MPP8–GLP interaction requires intact chromodomain of MPP8. HA-GLP–WT was coexpressed with Flag-MPP8-WT or its W80A mutant inMPP8stably knockdown 293T cells. Immunoprecipitation–western analyses were carried out using indicated antibodies. Methyl–lysine binding deficient MPP8 mutant W80A abrogates MPP8–GLP interaction in cells (comparing lanes 3 and 6). In, 5% input. (e) A hypothetical model of G9a/GLP–Dnmt3a-MPP8 complex mediated by generating and reading of methyl–lysine. A cartoon illustration of the proposed model of signalling cross-talk between the K44 methylated Dnmt3a, by the GLP component of the GLP/G9a heterodimer6, and recognized by the MPP8, resulting in a repressive chromatin with H3K9 methylation and DNA CpG methylation on chromatin templates. Figure 6: MPP8 binds self-methylated GLP. ( a ) GLP self-methylates lysine residue at K205. Wild-type (WT) or K205R mutated GST–GLP–N terminal fragment (residues 191–280) was incubated with (lanes 3–4) or without (lanes 1–2) His–GLP–SET domain (residues 955–1,298) for methylation assays. Auto-radiogram (right) shows methylation. ( b ) MPP8 binds to methylated GLP at K205 in vitro . GST–GLP–N–WT or its K205R mutant in the context of fragment 191–280 was incubated with His–GLP–SET domain for in vitro methylation. After being purified and immobilized on glutathione beads, GST–GLP–N terminal fragment was incubated with in vitro translated FL- 35 S–MPP8–WT (top panel) or its W80A mutant (bottom panel) for GST pull-down. Label 'B' indicates the bound fraction and 'Ft' the flow through. In, 5% input. ( c ) MPP8–GLP interaction is mediated through GLP–K205 in cells. Flag-MPP8-WT was coexpressed with HA-GLP–WT, K199R, K205R or K209R mutant in 293T cells. Cell lysates were immunoprecipitated with anti-HA (top panel) or Flag (bottom panel) antibody. Co-immunoprecipitated Flag-MPP8 or HA–GLP were analysed by western blot using indicated antibodies. In, 5% input. ( d ) MPP8–GLP interaction requires intact chromodomain of MPP8. HA-GLP–WT was coexpressed with Flag-MPP8-WT or its W80A mutant in MPP8 stably knockdown 293T cells. Immunoprecipitation–western analyses were carried out using indicated antibodies. Methyl–lysine binding deficient MPP8 mutant W80A abrogates MPP8–GLP interaction in cells (comparing lanes 3 and 6). In, 5% input. ( e ) A hypothetical model of G9a/GLP–Dnmt3a-MPP8 complex mediated by generating and reading of methyl–lysine. A cartoon illustration of the proposed model of signalling cross-talk between the K44 methylated Dnmt3a, by the GLP component of the GLP/G9a heterodimer [6] , and recognized by the MPP8, resulting in a repressive chromatin with H3K9 methylation and DNA CpG methylation on chromatin templates. Full size image Furthermore, co-immunoprecipitation of Flag-MPP8 and HA–GLP indicated K205R mutation of GLP impairs GLP–MPP8 interaction in cells whereas adjacent K199R or K209R mutation had little effect ( Fig. 6c ). Substitution of the cage residue Trp80 to Ala in the MPP8 chromodomain impaired MPP8–GLP interactions when they were coexpressed in MPP8 stable knockdown 293T cells ( Fig. 6d ). Additionally, no interaction was observed in GST pull-down assays between MPP8–W80A and WT, K205-methylated or K205R-mutated GLP–N ( Fig. 6b , bottom panel). Collectively, these results demonstrate that GLP–K205 self-methylation creates a binding site for MPP8 and directly mediates GLP–MPP8 protein–protein interaction. Dnmt3a and G9a/GLP catalyze, respectively, de novo DNA CpG methylation and histone H3K9 methylation, generating chromatin marks generally associated with transcriptional repression. For these signals to synergize, one enzyme needs to recruit the other to the same or nearby nucleosome(s). Dnmt3a was efficiently recruited to the silenced Oct3/4 promoter via its unique N-terminal domain during all-trans retinoic acid-induced mouse embryonic stem cell differentiation [27] . Here we show, enzymatically and structurally, that the N-terminal lysine K44 of mDnmt3a (or equivalent K47 of hDNMT3A) is methylated by GLP or G9a in vitro , and when GLP or G9a are overexpressed in cells. We suspect that GLP might be the primary protein lysine methyltransferase responsible for the mDnmt3a lysine 44 modification, because the enzymatic activity of G9a is more important for H3K9 methylation in vivo than that of GLP [19] , [26] . Whereas the GLP/G9a-mutant complex does not rescue global H3K9 methylation, the CpG sites of the promoter regions of G9a/GLP-target genes remain methylated in such mutant ES cells. One possible interpretation is that the GLP/G9a-mutant complex is still able to interact with Dnmt3a (via K44), thus carries out DNA methylation on target promoters (independent of H3K9 methylation) and suppresses transcription. We also show that the MPP8 chromodomain recognizes the dimethylated K44 of mDnmt3a (or K47me2 of hDNMT3A), with a binding affinity similar to that of HP1 chromodomain binding of H3K9me3 (ref. 43 ). MPP8 knockdown decreases DNA methylation in the 3′ region of E-cadherin CpG island attended by the loss of hDNMT3A localization, but does not affect GLP localization and H3K9 methylation patterns in the same region [24] . Additionally, hDNMT3A localization can be completely restored by rescue expression of MPP8-WT but not the cage mutant W80A [24] , which lost its ability to interact with hDNMT3A ( Fig. 4g ) and GLP ( Fig. 6b,d ). Interestingly, G9a and GLP are automethylated at their respective N-terminal regions [28] , [41] , [42] and the autocatalytic GLP methylation at K205 is also recognized by MPP8 ( Fig. 6 ). The potential formation of a dimeric MPP8 chromodomain in solution [44] as well as in crystals ( Supplementary Fig. S5 ) suggests that a MPP8 dimer could bridge the methylated Dnmt3a and GLP ( Fig. 6e ), resulting in a silencing complex of Dnmt3a–MPP8–GLP/G9a on chromatin templates. Together, our results reveal how the integration of multiple signals that establishes DNA methylation and H3K9 methylation at chromatin. A noteworthy observation is that the residue immediately after the target lysine is a valine in Dnmt3a and a threonine in GLP ( Fig. 1a ). The presence of a phosphorylatable threonine adjacent to K205 led us to speculate that phosphorylation on T206 could disrupt MPP8–GLP interaction in a manner analogous to the methylation–phosphorylation switch of K9-S10 of histone H3 (ref. 45 ), K142-S143 of DNMT1 (ref. 46 ) and K310-S311 of the NF-κB subunit RelA [39] . We also speculate that the chromodomain of another H3K9 methyltransferase Suv39h might interact with DNA methyltransferase Dnmt3b, because Suv39h contains a chromodomain within the same polypeptide [47] and there exists a physical and functional link between the Suv39h–HP1 histone methylation system and Dnmt3b [48] . Besides H3K9 methylation, histone H3 lysine 27 (H3K27) methylation has, in some instances, been demonstrated to crosstalk with de novo DNA methylation [49] . Components of the polycomb complex that either generate [50] or read [51] H3K27 methylation are associated with DNA methyltransferases. Together with our observations here, we hypothesize that dynamic posttranslational modifications of Dnmt3a, and possibly Dnmt3b and Dnmt1, might be a component of mechanism(s) to target this key epigenetic DNA methyltransferase to chromatin templates with appropriately histone modifications. Protein expression and purification All constructs were expressed in Escherichia coli BL21 (DE3) Codon-plus RIL (Stratagene) harbouring the RIL-Codon plus plasmid ( Supplementary Table S2 ). Expression was induced with 0.4 mM isopropyl β-D-thiogalactoside for 16 h at 16 °C in LB medium. Proteins were generally purified via three-column chromatography (GE Healthcare). For 6xHis–SUMO fusion protein (hMPP8 chromodomain), a HisTrap HP column was used to trap the fusion protein. Following imidazole elution, the 6xHis–SUMO tag was cleaved off by Ulp1 protease overnight, leaving two extraneous N-terminal amino acids (His-Met) fused to the target protein. The 6xHis–SUMO tag and the Ulp1 protease were removed by passing the mixture through the nickel column again. The protein was further purified by HiTrap Q and HiLoad Superdex 75 chromatography and stored in 20 mM Tris–HCl pH 8.0, 400 mM NaCl and 1 mM dithiothreitol. For N-terminal hexahistidine (6xHis) tagged protein (GLP SET domain), we isolated the protein on a HisTrap HP column. After imidazole elution, the 6xHis tag was cleaved by thrombin protease during overnight dialysis at 4 °C. Two extraneous N-terminal amino acids (Gly–Ser) were fused to the N-terminal residues. We further purified the protein by ion-exchange (HiTrap-Q) and gel filtration chromatography (Superdex-75 or -200). For GST-tagged fusion protein (mDnmt3a N-terminal fragment), we used a GST affinity column and while the fusion protein was still on the column, the GST-tagged proteins were cleaved with PreScission protease overnight ( ∼ 16 h) at 4 °C, and then further purified utilizing HiTrapSP and S75 or S200 Superdex sizing columns. For N-terminal Flag-tagged hDNMT3A full-length proteins (WT or K47R mutant), from 293T cells transfected with corresponding expression vectors, we purified the proteins using an antibody affinity column. Cells were lysated with IPH buffer (50 mM Tris–HCl, pH 8.0, 150 mM NaCl, 0.5% NP40) followed by micrococcal nuclease (Worthington) digestion and brief sonication. Cell lysates were incubated with anti-Flag (M2) agarose (Sigma) for immunoprecipitation. After washing three times with IPH buffer containing 1 M NaCl, immunoprecipitated proteins were eluted out using synthesized Flag-peptide. In vitro methylation assay A 20-μl reaction was carried out at 30 °C for 8 min in buffer of 20 mM Tris–HCl pH 8.5 with 2.8 μM [methyl- 3 H]AdoMet, 1.6 μM either hG9a or hGLP SET domain (in 20 mM Tris 8.0, 150 mM NaCl, 1 mM dithiothreitol) and 13.0 μM substrate (mDnmt3a and other proteins used in Supplementary Fig. S1 ). Samples were analysed by SDS–PAGE and fluorography. In vitro GST pull-down assay For in vitro GST pull-down, ∼ 3 μg of GST–hGLP–N (WT or K205R mutant) incubated with 3 μg 6xHis–hGLP–SET ( Fig. 6a ), respectively, in the presence of 1.5 mM AdoMet in a total 50-μl reaction at 30 °C for 2 h. The reaction was then incubated with 12 μl glutathione agarose and 50 μl buffer A (20 mM Tris–HCl, pH 7.6, 1 M NaCl, 0.2 mM EDTA, 1 mM DTT) for immobolization at 4 °C for 1 h, followed by washing with buffer A containing 0.1% NP40 and GST-binding buffer (10 mM Tris–Cl, pH 7.6, 150 mM NaCl, 1 mM MgCl 2 , 0.1% Triton-X 100, 5% glycerol, 1 mM dithiothreitol). The beads were next incubated with 5 μl of in vitro translated 35 S–MPP8–FL proteins (WT or W80A mutant) in 200 μl GST-binding buffer at 4 °C for 2 h. After washing with GST-binding buffer containing 300 mM NaCl three times and GST-binding buffer two times, bound proteins were analysed by SDS–PAGE autoradiography ( Fig. 6b ). 5% of in vitro translated 35 S–MPP8–FL applied for each binding assay was indicated as 'In' on autoradiography. Immunoprecipitations and binding assays 293T cells were transfected with different expression vectors in 10-cm dishes for 48 h and lysated with IPH buffer followed by brief sonication and micrococcal nuclease digestion to release chromatin-bound proteins. Immunoprecipitations were then carried out using 1 μg of mouse IgG, anti-Myc (9E10), anti-HA (12CA5) or anti-Flag (M2) together with 10 μl of protein-G agarose. After washing with IPH buffer containing 300 or 600 mM NaCl three times, immunoprecipitated proteins were subjected to SDS–PAGE and followed by western blot analysis. About 1–2 or 5% of cell lysates applied for each immunoprecipitation was indicated as 'In' on western blot analyses of MPP8–hDNMT3A or MPP8–GLP protein–protein interactions, respectively. In vivo metabolic labelling Briefly, myc-hDNMT3A was expressed with or without Flag-tagged GLP or G9a in GLP stable knockdown 293T cells for 36 h. After being starved for 30 min in methionine-free medium supplemented with cycloheximide (100 μg ml −1 ) and chloramphenicol (40 μg ml −1 ), transfected cells were labelled with 10 μCi ml −1 L -[methyl-3H]methionine (PerkinElmer) for 4 h. Myc-hDNMT3A was then immunoprecipitated with anti-Myc antibody (9E10) and extensively washed with IPH buffer containing 600 mM NaCl. The baseline signal in Figure 2a is very likely due to the incorporation of 3 H-Met in the methionine-free medium. MS analysis by MALDI–TOF Protein bands were stained with Coomassie blue using 17% SDS–PAGE gel. Protein bands of mDnmt3a N-terminal fragment (residue 1–274) were carefully excised, cut into small cubes and placed in a clean Eppendorf tube. The gel was washed 3 times with 10 mM ammonium bicarbonate, 50% acetonitrile, followed by a wash with 10 mM ammonium bicarbonate. The gel pieces were then dried in a speed vacuum and rehydrated with 5–10 μl of 10 mM ammonium bicarbonate containing 0.2–0.5 μg endoproteinase GluC, enough to cover the gel cubes. The samples were incubated at 37 °C overnight. Then they were centrifuged and added up to 1% TFA to stop the digestion. Removed supernatant and saved in a new Eppendorf tube. Remaining peptides were extracted using 100 μl 60% acetonitrile for 3 times. The extracts and the digestion solution were pooled and dried in speed vacuum until about 10 μl. For mass measurement ( Fig. 1c ), mixed 1 μl of the digestion sample with 1 μl saturated solution of a-cyano-4-hydroxycinnamic acid and spotted on a MTP 384 target plate. Mass was measured by MALDI–TOF in reflective mode on a Bruker Ultraflex II TOF/TOF instrument (Biochemistry Department, Emory University). MS analysis by LC–MS/MS Gel bands containing hDMNT3A were excised and destained. The disulfide bonds in the proteins were reduced with tris(2-carboxy-ethyl)phosphine; cysteines were reduced with iodoacetamide. Aliquots were digested with modified trypsin (Promega) in 30 mM ammonium bicarbonate, endoproteinase Glu-C (Roche) in 50 mM phosphate buffer, and endoproteinase Lys-C (Roche) in 25 mM Tris with 1 mM EDTA adjusted to pH 8.5. Trypsin and Glu-C digestions were performed overnight at 37 °C; Lys-C digestions were performed overnight at room temperature. Peptides were extracted from the gel and concentrated by vacuum centrifugation before analysis with LC–MS/MS. Peptide synthesis We synthesized peptides mDnmt3a(39–50)K44 SATAR K VGRPGR and hDNMT3A(39–53)K47 YEPSTTAR K VGRPGR (with underlined K in unmodified or dimethylated form) at the W.M. Keck Foundation Biotechnology Resource Laboratory (Yale University). The hDNMT3AK47 peptides were quantified by the absorbance of an added N-terminal tyrosine (residue 39), whereas the mDnmt3aK44 were quantified by weighing. Isothermal titration calorimetry measurements The isothermal titration calorimetry (ITC) experiments were conducted at 25 °C in 20 mM Tris–HCl pH 8.0, 150 mM NaCl. Protein concentrations were measured by absorbance spectroscopy at 280 nm. The titrations of mDnmt3a peptides against GLP or G9a were performed with a MicroCal VP–ITC instrument ( Fig. 3a ; Supplementary Fig. S4a ), and the titrations of hDNMT3A peptides against SUMO-tagged MPP8 were conducted with an Auto-iTC200 instrument (GE Healthcare) ( Fig. 4a ). The reference titration of corresponding peptide into SUMO alone was subtracted from experimental data. We calculated binding constants by fitting the data using the ITC data-analysis module of Origin 7.0 (OriginLab). The use of Auto-iTC200 is supported by award 104177 from the National Science Foundation, the Winship Cancer Institute and the Biochemistry Department of Emory University. Crystallography For crystallization of the GLP SET domain in complex with AdoHcy (or Sinefungin) and mDnmt3aK44me2 (or me0) peptide (residues 39–50), the purified protein (in 20 mM Tris 8.0, 400 mM NaCl) was incubated with cofactor analogue and peptide at 1:2:8 molar ratio on ice for 1 h. The final protein concentration is 23 mg ml −1 . Crystals were obtained by hanging-drop vapour-diffusion method at 16 °C after 1–2 days, with mother liquor containing 0.1 M HEPES, pH 7.5, 16% polyethylene glycol 4000 and 8% isopropanol. Crystals were flash-frozen in liquid nitrogen with mother liquor containing 20% glycerol. For crystallization of MPP8 chromodomain in complex with hDNMT3A-K47me2 peptide (residues 39–53), the purified protein was concentrated to about 40 mg ml −1 mixed with peptide at 1:1.5 molar ratio in buffer containing 20 mM Tris–HCl, pH 8.0, 400 mM NaCl and 1 mM tris(2-carboxy-ethyl)phosphine. Initial crystals were generated after 10 days by hanging-drop vapour-diffusion method, under the conditions of 30% polyethylene glycol 1500, 20% polyethylene glycol 400 and 0.1 M HEPES, pH 7.5. Better quality crystals were obtained under the same condition by micro-seeding within 2 days of setting up the crystallization drops. For data collection, the crystals were equilibrated in a cryoprotectant buffer containing reservoir solution plus 20% glycerol. The X-ray data were collected at the NE–CAT beamline 24-ID-C or SER–CAT beamlines 22-BM and 22-ID at the Advanced Light Source (APS), Argonne National Laboratory. Accession codes: The coordinates and structure factors have been deposited in the Protein Data Bank under accession codes 3SW9 (for GLP SET domain-mDnmt3aK44me0-Sinefungin), 3SWC (for GLP SET domain–mDnmt3aK44me2–AdoHcy) and 3SVM (for MPP8 chromodomain–hDNMT3AK47me2). How to cite this article: Chang, Y. et al . MPP8 mediates the interactions between DNA methyltransferase Dnmt3a and H3K9 methyltransferase GLP/G9a. Nat. Commun. 2:533 doi: 10.1038/ncomms1549 (2011).